Nanoscale visualization of redox activity at lithium-ion battery cathodes Intercalation and deintercalation of lithium ions at electrode surfaces are central to the operation of lithium-ion batteries. Yet, on the most important composite cathode surfaces, this is a rather complex process involving spatially heterogeneous reactions that have proved difficult to resolve with existing techniques. Here we report a scanning electrochemical cell microscope based approach to define a mobile electrochemical cell that is used to quantitatively visualize electrochemical phenomena at the battery cathode material LiFePO 4 , with resolution of ~100 nm. The technique measures electrode topography and different electrochemical properties simultaneously, and the information can be combined with complementary microscopic techniques to reveal new perspectives on structure and activity. These electrodes exhibit highly spatially heterogeneous electrochemistry at the nanoscale, both within secondary particles and at individual primary nanoparticles, which is highly dependent on the local structure and composition. Lithium-ion batteries have a remarkably wide range of applications from portable electronics to hybrid electric vehicles, where high energy, power and long-term cycling stability are in demand [1] . However, the rational development and improvement of battery technologies requires a better view of fundamental properties of redox activity at battery electrode surfaces. Although several techniques have been developed to visualize physicochemical processes in batteries and battery materials [2] , [3] , [4] , [5] , [6] , [7] , mapping redox activity of battery electrodes remains challenging owing to a lack of effective analytical tools, not least because battery electrodes are typically very rough on the microscale but show activity variations on the nanoscale. To address this issue, in this paper, we describe a powerful approach for visualizing redox activity at complex composite electrodes at high spatial resolution. Although electrochemical imaging via scanning electrochemical microscopy (SECM) can achieve high resolution in certain applications, such measurements are rare and tend to be applied to flat (topographically uninteresting) surfaces if activity is to be measured quantitatively [8] , [9] . Hitherto, microscopic understanding of the redox activity of the battery electrodes has relied on just a few techniques. A microelectrode–particle contact method has been used to evaluate the electrochemical processes at single active cathode electrode particles [10] , [11] , [12] , but the process was either measured for the whole grain (relatively large secondary particle) or, in special circumstances, information was obtained at a resolution of several microns (or larger) by using in situ optical or Raman visualization techniques [12] . At higher resolution, atomic force microscopy (AFM) and scanning tunneling microscopy (STM) have been used to visualize dynamic structural changes during charge/discharge, for instance, solid electrolyte interface formation [13] , [14] . More specialized scanned probe microscopes have proven particularly powerful for in situ high-resolution dynamic mapping, as exemplified by electrochemical strain microscopy [15] , [16] , [17] , [18] and scanning ion conductance microscopy [19] studies. For local dynamic electrochemical measurements, SECCM [20] , [21] , [22] , [23] , [24] , [25] and related techniques [26] appear particularly promising for direct, local electrochemical measurements, and we thus develop this platform herein to identify key processes underpinning the performance of battery electrodes. As a model system, but one that is also of practical importance, we study lithium iron phosphate (LiFePO 4 ) cathode materials, which have found application in both aqueous [27] , [28] , [29] and non-aqueous [10] , [30] electrolyte lithium-ion batteries. LiFePO 4 has attracted particular interest owing to its low cost, excellent safety profile and for environmental considerations. However, a drawback is that LiFePO 4 suffers from low electronic conductivity [31] , requiring that it is blended with a conductive material such as acetylene black (AB). This results in a complex composite material for which the local structure–function properties are largely unknown, and hence is considered as an ideal system to demonstrate the capabilities of SECCM imaging and multi-microscopy [32] . Here, we use single-channel SECCM to map spatial heterogeneities in the electrochemistry of LiFePO 4 electrodes, and to link these to local topography and surface chemistry using complementary imaging techniques. We attain a spatial resolution for electrochemical activity mapping that is more than two orders of magnitude better than the best resolution from previous (recent) electrochemical imaging studies of such materials [33] . We are also able to investigate the behaviour of individual pure LiFePO 4 primary nanoparticles for the first time. This enables us to identify key factors controlling electrochemistry and (de)intercalation, from elementary nanomaterials to whole device electrodes. 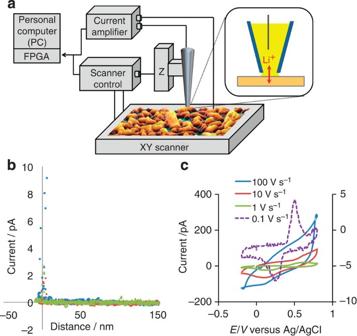Figure 1: Experimental overview and local electrochemical measurements. (a) Schematic of the SECCM. (b) Approach characteristics (current–distance) for three different nanopipettes (3 M LiCl) moved towards a LiFePO4electrode with a bias voltage of +0.65 V versus Ag/AgCl QRCE. (c) CVs obtained with nanopipette meniscus contact (3 M LiCl) at different scan rates on a LiFePO4electrode. CV with 0.1 V s−1uses the right axis and the other CVs use the left axis. Localized electrochemical measurements Figure 1a is a schematic of single-channel SECCM that allows us to visualize and measure various electrochemical properties simultaneously with electrode topography. The principles and operation of the technique are similar to those outlined elsewhere [26] , but we use a 50-nm radius nanopipette in a hopping mode to obtain high spatial resolution electrochemical images, even on a very rough electrode surface. Moreover, we explore new modes for meniscus-based imaging, such as zero-current (essentially open circuit) cell potential mapping and local charge/discharge modification. Figure 1: Experimental overview and local electrochemical measurements. ( a ) Schematic of the SECCM. ( b ) Approach characteristics (current–distance) for three different nanopipettes (3 M LiCl) moved towards a LiFePO 4 electrode with a bias voltage of +0.65 V versus Ag/AgCl QRCE. ( c ) CVs obtained with nanopipette meniscus contact (3 M LiCl) at different scan rates on a LiFePO 4 electrode. CV with 0.1 V s −1 uses the right axis and the other CVs use the left axis. Full size image The technique uses a moveable nanopipette probe (typical radius of 50 nm; Supplementary Note 1 and Supplementary Fig. 1 ) usually containing 3 M LiCl electrolyte solution and an Ag/AgCl quasi-reference counter electrode (QRCE). The nanopipette was brought into close contact with a sample electrode surface via a liquid meniscus at the nanopipette end. For initial experiments, the sample LiFePO 4 composite electrode was connected to a current amplifier and a bias voltage of +0.65 V versus Ag/AgCl QRCE was applied with the QRCE connected to ground. The cell current versus probe (meniscus) to sample separation is shown in Fig. 1b for three different nanopipettes approached towards the surface at 20 nm ms −1 . When the meniscus just made contact with the surface, a small anodic current flowed and a set point of 2 pA triggered the nanopipette to stop from further approaching. During imaging, the tip height position at this point was recorded, enabling the topography of the surface to be tracked. Localization of the electrochemical cell to the footprint of the meniscus allowed the LiFePO 4 charge/discharge reaction to be probed at the nanoscale without the LiFePO 4 electrode being completely immersed in solution. The redox reaction of interest is: with the process left to right corresponding to discharge (Li + intercalation), which is a main focus of the studies herein. Major advantages of our approach are that working electrode/electrolyte interface can be created at defined locations via a moveable nanopipette, and the nanoscale footprint of the electrochemical cell diminishes ohmic effects and capacitive currents during electrochemical measurements and imaging. Figure 1c shows examples of cyclic voltammograms (CVs) on a LiFePO 4 thin-film electrode. The working electrode potential was linearly ramped up from 0 to 0.8 V, returned to −0.2 V and then scanned back to 0 V versus Ag/AgCl (scan rates in the range 0.1 to 100 V s −1 ). At 0.1 V s −1 , there is a clear anodic peak at ca. 0.49 V (at 0.1 V s −1 ) corresponding to the oxidation of Fe II to Fe III with deintercalation of Li + . Upon reversing the potential, the reverse process (Fe III reduction to Fe II , with Li + intercalation) occurs at ca. 0.27 V. The peak-to-peak separation is similar to that measured at the same timescale on LiFePO 4 microelectrodes [34] , confirming the validity of our new approach, which is most powerfully used for imaging as discussed next. The (de)intercalation process is quasi-reversible [30] , as evidenced by the peak-to-peak separation increasing further with increasing scan rate in the range 1–100 V s −1 . The upper value is the fastest voltammetric timescale applied to LiFePO 4 redox activity and (de)intercalation by two orders of magnitude [34] , and it is clear that the transformation is reasonably facile. Note that when the solution in the nanopipette was replaced with one containing 3.0 M KCl, negligible redox activity and (de)intercalation was observed ( Supplementary Note 2 and Supplementary Fig. 2 ). Electrochemical imaging of composite LiFePO 4 electrodes In this section, we highlight major capabilities of SECCM in visualizing redox activity at high spatial resolution and linking this to topography and surface chemistry at the nanoscale. We also demonstrate the measurement of charge–discharge curves at desired nanoscale locations and carry out surface potential measurements to allow ‘chemical’ mapping (identification of LiFePO 4 domains). We further show how SECCM allows the charge state of a complex electrode to be changed and visualized locally, opening up the manipulation of the electrode surfaces and new measurement possibilities. First, a secondary electroactive particle ( ϕ =3 μm) of LiFePO 4 , attached with poly(vinylidenedifluoride) (PVdF) binder and AB in a composite electrode, was measured. 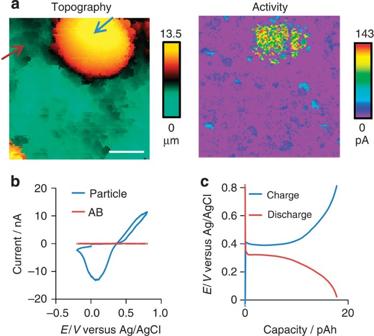Figure 2: Topography and current activity of a LiFePO4electrode. (a) Simultaneous SECCM topography (left) and current (right) images. Scan ranges are 20 × 20 μm. The substrate potential was +0.65 V versus Ag/AgCl QRCE (Li+deintercalation; scale bar, 5 μm). (b) CVs at different points on a LiFePO4electrode surface, corresponding to the blue and red arrow ofb. Scan rate is 0.1 V s−1. (c) Local charge (deintercalation) and discharge (intercalation) characteristics applying current magnitudes of 200 pA in each case via SECCM. Figure 2b shows typical topography and interfacial current images obtained simultaneously by SECCM, with the electrode potential at +0.65 V (just into the Li + deintercalation process; Fig. 1c ). Notably, a high current response was observed at the location of the mound in the region probed. This topographical feature can reasonably be assigned as a secondary particle based on Scanning Electron Microscope (SEM)–energy dispersive X-ray spectroscopy (EDS) images of a typical electrode area and the fact that there is excellent correspondence of the current and particle position maps, with little current flow elsewhere. Importantly, however, although the secondary particle (comprising primary particles of different orientation) can be identified, it is also clear that within the particle the redox activity is highly heterogeneous. We consider the origin of this further below, when examining individual primary nanoparticles. As shown in Supplementary Note 3 and Supplementary Fig. 3 , rates (currents) of the intercalation and deintercalation processes are strongly spatially correlated across a LiFePO 4 electrode surface. Figure 2: Topography and current activity of a LiFePO 4 electrode. ( a ) Simultaneous SECCM topography (left) and current (right) images. Scan ranges are 20 × 20 μm. The substrate potential was +0.65 V versus Ag/AgCl QRCE (Li + deintercalation; scale bar, 5 μm). ( b ) CVs at different points on a LiFePO 4 electrode surface, corresponding to the blue and red arrow of b . Scan rate is 0.1 V s −1 . ( c ) Local charge (deintercalation) and discharge (intercalation) characteristics applying current magnitudes of 200 pA in each case via SECCM. Full size image After imaging, the nanopipette was positioned to make meniscus contact at locations corresponding to the particle (blue arrow in Fig. 2a ) and away from the particle (red arrow) to enable localized CV measurements ( Fig. 2b ). Significant redox activity and (de)intercalation was observed on the particle, confirming the correlation of the current with the position of LiFePO 4 . Away from the particle, only a very weak current–voltage response was observed, suggesting that this was an area of AB. SECCM also allowed charge/discharge characteristics to be determined on secondary particles within a composite electrode ( Fig. 2c ). Here a current magnitude of 200 pA was applied via nanoscale meniscus contact, and the potential–time curves for charge and discharge were recorded. There is excellent correspondence of the morphology of two curves, from which the capacity was estimated to be ~15 pA h. The reacted volume is ~25 μm 3 using theoretical volumetric capacity (612 mA h cm −3 ), corresponding to a spherical radius of 1.8 μm. This is about the same size of a small secondary particle, such as that in Fig. 2c . Thus, this analysis indicates that individual secondary particles within a LiFePO 4 composite electrode can be targeted and characterized by local electrolyte contact, without influence from neighbouring particles. Potential imaging of composite LiFePO 4 electrodes We now demonstrate SECCM as a powerful technique for local potential mapping. The condition of this measurement was zero current in an electrochemical cell (applied after landing a meniscus at each point on the surface investigated), so that a potential close to an open circuit value was measured, as described in the experimental section. 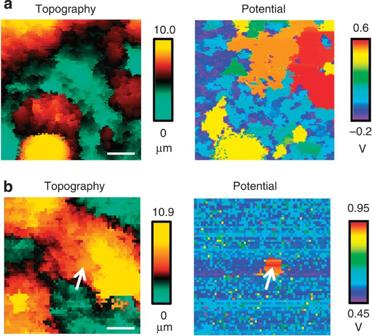Figure 3: Topography and potential images of a LiFePO4electrode. (a) Simultaneous SECCM topography (left) and potential (right) images (15 × 15 μm; scale bar, 3 μm). (b) Simultaneous SECCM topography (left) and surface potential (right) images after charging the electrode (Li+deintercalation) locally at a point on the electrode (until the potential reached +0.8 V; scale bar, 5 μm). Images are 25 × 25 μm. The white arrow shows the charging point on the topography and potential map. Figure 3a shows an example of cell potential mapping of a LiFePO 4 film with AB and PVdF binder. A highly spatially inhomogeneous potential can be seen. Regions where the value is ca. +0.4~0.6 V can be assigned to LiFePO 4 , based on the redox potential for Li + (de)intercalation (for example, Fig. 1c ). In other regions, it was difficult to achieve a steady potential. We attribute these to AB regions that would show behaviour close to that of an ideally polarizable electrode [35] . The SECCM data in this two-component system indicate that potential mapping is powerful for highlighting different types of material in a composite electrode. Figure 3: Topography and potential images of a LiFePO 4 electrode. ( a ) Simultaneous SECCM topography (left) and potential (right) images (15 × 15 μm; scale bar, 3 μm). ( b ) Simultaneous SECCM topography (left) and surface potential (right) images after charging the electrode (Li + deintercalation) locally at a point on the electrode (until the potential reached +0.8 V; scale bar, 5 μm). Images are 25 × 25 μm. The white arrow shows the charging point on the topography and potential map. Full size image We were also able to change the local redox state (Li + concentration) in the LiFePO 4 by inducing the deintercalation reaction using nanopipette meniscus contact and by imaging the resulting cell potential distribution. For these measurements, the nanopipette meniscus was positioned at the centre of the sample surface and localized charging was performed (+200 pA) until the voltage reached 0.8 V (taking ca. 1 h). The cell potential was then mapped, yielding the image in Fig. 3b . At the centre of the LiFePO 4 (white arrow), there is a higher potential (~0.8 V) at the position where the oxidation of Fe II to Fe III (Li + deintercalation) occurred, highlighting that the local redox state and composition in LiFePO 4 can be manipulated with high control. This local perturbation approach might be usable in the future to probe solid state diffusion coefficients, among other applications. Local galvanostatic charge/discharge property mapping To further demonstrate charge/discharge imaging and to highlight unequivocally how this linked to the chemical character of a composite electrode, localized charging was performed (+5.0 pA) for 600 ms (total charge 3 fC) at each measurement point, with the potential–time characteristic measured simultaneously (10 ms time resolution). The 3 fC charge corresponds to a spherical radius of ca. 57 nm based on the LiFePO 4 theoretical volumetric capacity (612 mA h cm −3 ), ensuring that this measurement was surface sensitive. We further visualized the same region of the LiFePO 4 thin film by SEM–EDS to allow the unambiguous identification of LiFePO 4 particles from the strong oxygen signal ( Fig. 4a ). To enable different microscopies to be applied to the same region of the sample, we focused on a region near the edge of the LiFePO 4 thin film; the unique microscale topography of the sample allowed distinct features to be used for co-location of the different microscopy techniques. Particles evidently appear as small (micron scale) mounds in the surface (as proposed for the analysis of Fig. 2a ); compare the morphologies obtained by different techniques in Fig. 4a,b . 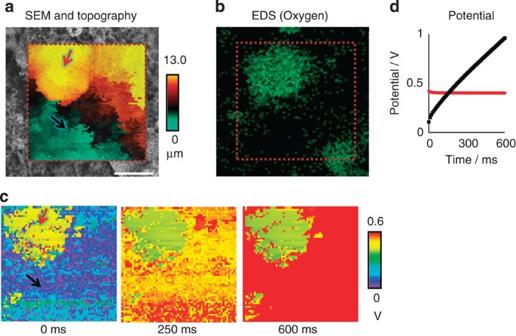Figure 4: Galvanostatic charge property mapping. (a) SEM and topography overlap image of a LiFePO4electrode (scale bar, 10 μm). (b) EDS (oxygen) image of the same area. (c) Potential images at times of 0, 250 and 600 ms (30 × 30 μm) during galvanostatic charging at +5.0 pA. (d) Galvanostatic potential–time curves at pixels on (red) and off (black) a secondary LiFePO4particle. Figure 4: Galvanostatic charge property mapping. ( a ) SEM and topography overlap image of a LiFePO 4 electrode (scale bar, 10 μm). ( b ) EDS (oxygen) image of the same area. ( c ) Potential images at times of 0, 250 and 600 ms (30 × 30 μm) during galvanostatic charging at +5.0 pA. ( d ) Galvanostatic potential–time curves at pixels on (red) and off (black) a secondary LiFePO 4 particle. Full size image By acquiring potential–time data at each pixel, the resulting data can be the most powerful represented as a potential–time movie ( Supplementary Movie 1 ), with several snapshots shown in Fig. 4c . At the secondary LiFePO 4 particle, there is good correlation between the SECCM potential and LiFePO 4 particle, which is identified by oxygen (from phosphate) in the EDS image. At the centre of the secondary LiFePO 4 particle (red arrow), the potential is essentially fixed at 0.40 V on this timescale (consistent with the data in Fig. 2c ). This is also seen clearly in the potential–time plot in Fig. 4d from a pixel indicated by the red arrows in Fig. 4a,c . In contrast, away from the secondary particle, which can reasonably be considered as an AB area (black arrow), the potential did not reach steady state because of its polarizable property ( Fig. 4d ). To illustrate the relationship between potentiostatic redox activity and galvanostatic charge activity, we carried out both types of measurements in the same area of the LiFePO 4 composite electrode ( Supplementary Note 4 and Supplementary Fig. 4 ). Evidently, the stable potential-response area corresponds with the area of high current, which in turn has been shown to be a LiFePO 4 particle from topographical imaging and EDS mapping. These results mean that we are able to link the surface component (LiFePO 4 secondary particle or AB) and function (charge/discharge) unequivocally and unambiguously via a multi-microscopy approach in which SECCM is a central technique. Single LiFePO 4 nanoparticle imaging Finally, we investigated individual primary LiFePO 4 nanoparticles dispersed on a Pt substrate ( Fig. 5a ). This presented a heterogeneous substrate at two levels: first, the nanopipette meniscus mainly landed on a Pt substrate and only a small charging current was measured; second, even when the nanopipette located an LiFePO 4 nanoparticle, Li + deintercalation current (electrode potential +0.65 V) would depend on the orientation of the nanoparticle. Thus, a distinct inhomogeneity of the current, linked to the topography (nanoparticle height), measured by SECCM in hopping mode ( Fig. 1b ), was observed ( Fig. 5b ). The topographical image reveals the nanoparticle size distribution ( Fig. 5c ). The lowest currents (<10 pA), which comprise ca. 98% of the sampled surface, are mainly owing to the Pt substrate, whereas the broad current distribution at higher values can be attributed to the LiFePO 4 nanoparticles that are reasonably expected to have different crystal orientations [36] and phases [37] . This result ties closely to the activity images of secondary particles, discussed above (for example, Fig. 2b ), in which a broad range of reaction rates within a particle was found, which appears to be owing to different orientations of the primary nanoparticles, from which the secondary particles are composed. In the future, it should be possible to visualize any influence of grain orientation on redox activity and (de)intercalation kinetics, enabling optimum crystal structures and orientations to be identified. 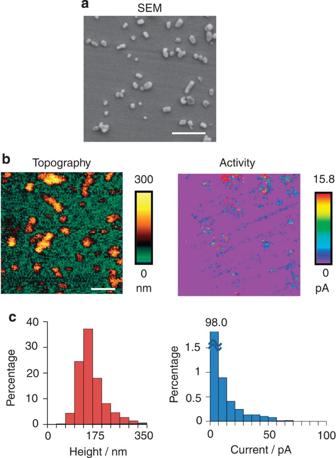Figure 5: Characterizing the activity and topography of individual LiFePO4nanoparticles. (a) SEM image of LiFePO4nanoparticles on a Pt collector electrode (scale bar, 1 μm). (b) Simultaneous SECCM topography (left) and current (right) images. Scan range is 5 × 5 μm (scale bar, 1 μm). The substrate potential was 0.65 V versus Ag/AgCl QRCE. (c) Data from the SECCM images of height (left), equivalent to particle size, and current (right), equivalent to deintercalation rate, plotted as histograms. Figure 5: Characterizing the activity and topography of individual LiFePO 4 nanoparticles. ( a ) SEM image of LiFePO 4 nanoparticles on a Pt collector electrode (scale bar, 1 μm). ( b ) Simultaneous SECCM topography (left) and current (right) images. Scan range is 5 × 5 μm (scale bar, 1 μm). The substrate potential was 0.65 V versus Ag/AgCl QRCE. ( c ) Data from the SECCM images of height (left), equivalent to particle size, and current (right), equivalent to deintercalation rate, plotted as histograms. Full size image In this paper, we have proposed a novel single-channel nanopipette SECCM method for the detailed characterization of Lithium-ion battery cathode materials. We have been able to map localized redox activity on LiFePO 4 composite electrode surfaces at the nanoscale for the first time, identifying significant variations in reaction rates that depend on local composition. Furthermore, local charging/discharging at LiFePO 4 particles in composite electrodes reveals that such processes are largely limited to the particle where the perturbation is made. This provides an opportunity to probe single particles and agglomerates in situ in complex composite materials, and to develop an understanding of how structure and function are related in complex composite battery electrodes. Importantly, where comparisons can be made with previous measurements, good agreement has been found, thereby giving confidence in the new insights obtained from this new local technique. We have highlighted the versatility of SECCM by mapping the open circuit potential of LiFePO 4 electrodes at the nanoscale and inducing charge/discharge processes locally. We have further been able to chemically map LiFePO 4 electrodes (identifying LiFePO 4 and AB domains from the cell potential response) and modify nanoscopic portions of macroscopic electrodes, opening up new measurement possibilities. The correlation of potential maps and current activity images with the underlying chemical composition of LiFePO 4 composite surfaces highlights the considerable strength of multi-microscopy measurements in understanding the structure and function of complex materials at the nanoscale. Finally, to further understand LiFePO 4 activity, we have been able to target primary nanoparticles and determine the distribution of electrochemical activity of such particles. A broad range of activity has been observed that links to the wide range of electrochemical fluxes seen across secondary particles, which comprises an agglomeration of such primary nanoparticles. This part of the study provides a foundation for future work, where it should be possible to determine how the orientation of crystallites influences electrochemistry and ion fluxes. Preparation of LiFePO 4 thin-film electrodes Both primary and secondary particles of LiFePO 4 were examined in this study. The procedure for synthesizing LiFePO 4 particles was described previously [38] . Primary particles were nanocrystals with a characteristic dimension of 100–200 nm that were non-carbon coated and dispersed onto a Pt current collector, which served as a specimen electrode. Test electrodes to examine secondary LiFePO 4 particles were prepared by a conventional method [30] in which a slurry of LiFePO 4 , AB (conductive agent) and PVdF (binder) was coated on an Al current collector using a doctor blade. N-methylpyrrolidone was used as a solvent for the slurry. The mixing ratio of LiFePO 4 :AB:PVdF was 92:4:4. The resulting secondary particle size was typically in the range of ~1–5 μm. Instruments The design of the instrument was similar to related electrochemical probe microscopes as previously described [39] , [40] , [41] , [42] . The current was measured by a dual-channel MultiClamp700B patch-clamp amplifier (Axon Instruments). The current signal during imaging was typically filtered using a low-pass filter at 1 kHz, except for CV at scan rates >1 V s −1 , where a 10-kHz low-pass filter was used. The data were digitized and analysed with continuous data acquisition hardware and software (Axon Digidata 1322A, Axon Instruments). The relative sample and probe position was precisely controlled by mounting the sample on an XY piezoelectric translation stage and the nanopipette on a Z stage (Nanocontrol, 621.2CL and 621.ZCL), both controlled by an amplifier module (Nanocontrol, NC3301). The system was controlled and data were acquired using LabVIEW (National Instruments). As well as being enclosed in a Faraday cage, the instrument was also enclosed in an acoustic isolation box (VIC International, VSD BM-1). The vertical Z positioning of the nanopipette and the movement of the sample in the XY plane were controlled (and recorded) by a Field Programmable Gate Array (FPGA) board (PCIe-7841R, National Instruments). SEM–EDS analysis was carried out with a Field Emission-Scanning Electron Microscope (FE-SEM) (JSM-7800 F, JEOL) and Energy Dispersive X-ray Spectrometer (Oxford Instruments, X-Max Silicon Drift Detector). Scanning protocol The following procedure was used to bring the nanopipette towards the sample surface so that the liquid meniscus just made contact (without contact from the nanopipette itself) at a series of predefined positions, with an electrochemical measurement at each point. First, the nanopipette (meniscus) was withdrawn from its existing position by a specified distance, typically 4.0 μm. Next, the vertical position of the probe was maintained for 20 ms, while the nanopositioning stage moved the specimen to a new imaging point in the xy plane. Then, the nanopipette was lowered at constant fall rate of 20 nm ms −1 while monitoring the current. Immediately after detecting a current (2 pA threshold) by forming the electrical contact between the nanopipette and the sample through the nanopipette meniscus, the approach was stopped and the vertical position of the nanopipette was saved along with the x,y co-ordinate to form a topography map. Twenty milliseconds then elapsed before the Li + (de)intercalation current was measured (50 μs duration, averaging 10 samples at a sampling frequency of 200 kHz). After the electrochemical measurement, the nanopipette was quickly withdrawn by the specified distance to start a new measurement cycle. In this way, simultaneous pictures of topography and redox activity were built up. Local cell potential mapping was performed by controlling the applied voltage so as to maintain the current from the sample working electrode to be zero by using the function of MultiClamp700B constant current mode. Fabrication of nanopipettes Nanopipettes were fabricated by pulling a borosilicate glass pipette (inner diameter=1.00 mm and outer diameter=0.78 mm; GC150F-10, Harvard Apparatus) using a laser puller (Sutter Instruments, model P-2000), with a two-step protocol. For the initial step, the parameters were heat 350, filament 3, velocity 21 and delay 200. The second step, they were heat 350, filament 2, velocity 26, delay 160 and pull 250. How to cite this article : Takahashi, Y. et al. Nanoscale visualization of redox activity at lithium-ion battery cathodes. Nat. Commun. 5:5450 doi: 10.1038/ncomms6450 (2014).